The lncRNA landscape of breast cancer reveals a role for DSCAM-AS1 in breast cancer progression Molecular classification of cancers into subtypes has resulted in an advance in our understanding of tumour biology and treatment response across multiple tumour types. However, to date, cancer profiling has largely focused on protein-coding genes, which comprise <1% of the genome. Here we leverage a compendium of 58,648 long noncoding RNAs (lncRNAs) to subtype 947 breast cancer samples. We show that lncRNA-based profiling categorizes breast tumours by their known molecular subtypes in breast cancer. We identify a cohort of breast cancer-associated and oestrogen-regulated lncRNAs, and investigate the role of the top prioritized oestrogen receptor (ER)-regulated lncRNA, DSCAM-AS1 . We demonstrate that DSCAM-AS1 mediates tumour progression and tamoxifen resistance and identify hnRNPL as an interacting protein involved in the mechanism of DSCAM-AS1 action. By highlighting the role of DSCAM-AS1 in breast cancer biology and treatment resistance, this study provides insight into the potential clinical implications of lncRNAs in breast cancer. Long noncoding RNAs (LncRNAs) have recently been implicated in a variety of biological processes, including carcinogenesis and tumour growth [1] , [2] , [3] , [4] , [5] , [6] . Operating through a myriad of mechanisms [2] , lncRNAs have challenged the central dogma of molecular biology as prominent functional RNA molecules. To investigate the role of lncRNAs in breast cancer, we interrogated the expression of lncRNAs across an RNA-sequencing (RNA-seq) breast tissue cohort comprised of 947 breast samples [7] , [8] . Previously, in a large-scale ab initio meta-assembly study from 6,503 RNA-seq libraries, we discovered ∼ 45,000 of unannotated human lncRNAs [7] , and this assembly was utilized for the present study. Building on prior work that has begun to investigate the role of lncRNAs in breast cancer [9] , we set out to perform a comprehensive analysis of breast cancer tissue RNA-seq data to identify the lncRNAs potentially involved in breast cancer. Patients with oestrogen receptor (ER)-positive breast cancer have better prognosis than those with ER-negative disease, based on both a more indolent natural history but perhaps more importantly due to effective anti-oestrogen, also designated ‘endocrine,’ therapy [10] . Despite the efficacy of endocrine therapy, however, the majority of breast cancer deaths occur in women with ER-positive breast cancers, because the incidence of ER-positive versus-negative disease is much higher (approximately 80 versus 20%), and because a substantial fraction of women either have inherent or acquired endocrine therapy-resistant disease [11] . Taken together, these considerations highlight the pressing need to understand the biology of the ER-driven breast cancers and their mechanism of resistance to endocrine therapy. The mechanism through which ER mediates cancer initiation and progression is an area of intense scientific investigation [12] , [13] , [14] that remains incompletely understood. In this regard, while substantial research has been focused on ER abnormalities, such as mutations in the gene encoding for ER ( ESR1 ) [14] , [15] and on the co-existing activation pathways that might mediate resistance, such as HER2 [16] , few studies exist that interrogate ER-regulated noncoding RNAs [17] , [18] , [19] , [20] , [21] . Therefore, we set out to perform a comprehensive discovery and investigation of those lncRNAs that are driven by oestrogen in breast cancers drawing from a large human tissue RNA-seq cohort. Identification of ER- and breast cancer-associated lncRNAs We initially focused on those lncRNAs most differentially expressed in breast cancers in comparison to benign adjacent tissue ( Supplementary Data 1 ), utilizing a non-parametric differential expression tool for RNA-seq called Sample Set Enrichment Analysis (SSEA) [7] . After applying an expression filter (at least one fragments per kilobase of transcript per million mapped reads (FPKM) expression in the breast samples in the top 5% based on gene expression level), we identified 437 of the most differentially expressed lncRNAs in breast cancer ( Supplementary Data 2 ). Interestingly, unsupervised hierarchical clustering of the samples based on expression of these lncRNAs across all breast cancer samples (Methods section) largely separated out the breast cancer samples by PAM50 subtypes [22] , [23] , suggesting that lncRNAs may be contributing to the distinct biology of these subtypes ( Fig. 1a ). While lncRNA expression was unable to distinguish between the ER-driven luminal A and luminal B subtypes, the luminal subtypes were well separated from the HER2, basal and normal subtypes ( Fig. 1a ). In addition to separating out the clinical subtypes of breast cancer, the lncRNAs themselves separated into three distinct clusters. The first cluster ( Fig. 1a , ‘Luminal’) contains lncRNAs overexpressed mostly in luminal A and luminal B samples, with little expression in samples of the other subtypes, and little expression in normal samples. The next cluster contains lncRNAs upregulated across all breast cancer samples ( Fig. 1a , ‘Upregulated’), and this cluster included the known breast cancer lncRNA, HOTAIR. The third cluster ( Fig. 1a , ‘Downregulated’) contains lncRNAs downregulated in breast cancers. The lncRNAs in the luminal cluster present a particularly intriguing class of potentially oestrogen-responsive lncRNAs. 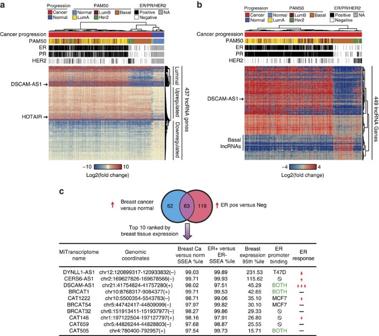Figure 1: Identification of ER and breast cancer-associated lncRNAs. (a) Heatmap depiction of the top cancer versus normal differentially expressed lncRNAs among the TCGA breast RNA-seq cohort (n=946). 437 lncRNAs were differentially expressed with an SSEA FDR<1e-5 and an SSEA percentile cutoff of 0.975 (Methods section). Expression values are depicted as log2 of the fold change over the median of the normal samples (n=104). Unsupervised hierarchical clustering was done on both lncRNAs and patients. Cancer progression, PAM50 classification, and ER, PR, and HER2 status are shown above heatmap. LncRNAs clustered into 3 distinct categories, ‘Luminal’, ‘Upregulated’, and ‘Downregulated’. Two representative lncRNAs are highlighted. (b) Heatmap depiction of the top ER-positive versus ER-negative lncRNAs. 449 lncRNAs met the SSEA criteria described ina. Unsupervised clustering was performed for samples and lncRNAs. Expression values depicted as log2 of the fold change over the median of the ER-negative samples (n=538). Cancer progression, PAM50 classification, and ER, PR and HER2 status are shown above heatmap. One representative lncRNA is highlighted along with a group of lncRNAs with basal-specific expression. (c) Venn diagram of the intersection of the breast cancer versus normal and ER-positive versus ER-negative analyses. Intersection is shown for the overexpressed lncRNAs in both categories. The top 10 lncRNAs based on expression level in breast cancer tissues (expression value of 95th percentile sample) are depicted in table. ER promoter binding determined via ChIP-seq is depicted (in either MCF7, T47D cell lines, or both) along with expression response from RNA-seq following 3 h of oestrogen stimulation in MCF7 cells (one arrow represents >1.5 fold increase, three arrows represents >2.5 fold increase). Figure 1: Identification of ER and breast cancer-associated lncRNAs. ( a ) Heatmap depiction of the top cancer versus normal differentially expressed lncRNAs among the TCGA breast RNA-seq cohort ( n =946). 437 lncRNAs were differentially expressed with an SSEA FDR<1e-5 and an SSEA percentile cutoff of 0.975 (Methods section). Expression values are depicted as log2 of the fold change over the median of the normal samples ( n =104). Unsupervised hierarchical clustering was done on both lncRNAs and patients. Cancer progression, PAM50 classification, and ER, PR, and HER2 status are shown above heatmap. LncRNAs clustered into 3 distinct categories, ‘Luminal’, ‘Upregulated’, and ‘Downregulated’. Two representative lncRNAs are highlighted. ( b ) Heatmap depiction of the top ER-positive versus ER-negative lncRNAs. 449 lncRNAs met the SSEA criteria described in a . Unsupervised clustering was performed for samples and lncRNAs. Expression values depicted as log2 of the fold change over the median of the ER-negative samples ( n =538). Cancer progression, PAM50 classification, and ER, PR and HER2 status are shown above heatmap. One representative lncRNA is highlighted along with a group of lncRNAs with basal-specific expression. ( c ) Venn diagram of the intersection of the breast cancer versus normal and ER-positive versus ER-negative analyses. Intersection is shown for the overexpressed lncRNAs in both categories. The top 10 lncRNAs based on expression level in breast cancer tissues (expression value of 95th percentile sample) are depicted in table. ER promoter binding determined via ChIP-seq is depicted (in either MCF7, T47D cell lines, or both) along with expression response from RNA-seq following 3 h of oestrogen stimulation in MCF7 cells (one arrow represents >1.5 fold increase, three arrows represents >2.5 fold increase). Full size image Using the 947 breast tumour RNA-seq samples ( Supplementary Data 1 ), we identified lncRNAs differentially expressed in ER-positive versus ER-negative breast tumours ( Fig. 1b , Supplementary Data 2 ). As expected, the expression of lncRNAs differentially expressed in ER-positive tumours separated the luminal tumours from the basal and HER2 on unsupervised hierarchical clustering ( Fig. 1b ). Quite interestingly, a number of lncRNAs that were downregulated in ER-positive samples exhibited increased expression in the basal samples ( Fig. 1b , ‘Basal lncRNAs’). While these basal lncRNAs were identified in an ER-positive versus ER-negative cancer analysis, a number of them also exhibit low expression in normal breast tissue ( Supplementary Fig. 1 ). Given that a paucity of known driver genes exist for basal breast cancers and that these tumours are the most clinically aggressive, these basal-specific lncRNAs may represent an exciting future area for basal breast cancer biology. We set out to investigate potentially oncogenic ER-regulated lncRNAs by intersecting the lncRNAs upregulated in both the cancer versus normal ( Fig. 1a ) and ER-positive versus ER-negative ( Fig. 1b ) analyses. Sixty-three lncRNAs were upregulated in both the cancer versus normal analysis and the ER-positive versus ER-negative analysis ( Supplementary Data 2 , Fig. 1c ). To prioritize the most biologically and clinically relevant lncRNAs, we focused on lncRNAs most highly expressed in breast cancer tissues, and those most directly regulated by ER, based on ER binding to the targets’ promoter as well as the degree of induction of expression following oestrogen stimulation in breast cancer cells ( Fig. 1c and Supplementary Fig. 2a ). This approach nominated DSCAM-AS1 as a lncRNA expressed at a very high level in breast cancer tissues, containing ER promoter binding, and exhibiting the strongest oestrogen induction in MCF7 and T47D cells by both RNA-seq and quantitative PCR (qPCR) validation ( Fig. 1c and Supplementary Fig. 2a ). We thus selected DSCAM-AS1 for further investigation. Characterization of DSCAM-AS1 DSCAM-AS1 has been previously reported to be involved in the proliferation of a luminal breast cancer cell line [20] . It exhibits a highly cancer-specific expression pattern, mostly in breast cancer and lung adenocarcinoma, in transcriptome sequencing data from a cohort of 6,503 cancer and normal tissues and cell lines from the TCGA and the Michigan Center for Translation Pathology [7] ( Fig. 2a ). Supporting its association with ER biology, DSCAM-AS1 expression is highly enriched (Student’s t -test, P value<10E −5 ) in ER-positive tumours among the breast cancer samples in this RNA-seq cohort with ER status determined by IHC ( Fig. 2b and Supplementary Data 1 ). In addition, analysis of RNA-seq performed on 50 breast cancer cell lines [24] revealed that expression of DSCAM-AS1 is highly specific to ER-positive cell lines ( Fig. 2c and Supplementary Fig. 2b ). Further supporting the association of ER with DSCAM-AS1 , ER chromatin immunoprecipitation-sequencing (ChIP-seq) in both MCF7 and T47D identified ER binding to the DSCAM-AS1 promoter following oestrogen stimulation ( Fig. 2d ), and this finding was confirmed by ChIP-qPCR of the DSCAM-AS1 promoter ( Supplementary Fig. 2c ). The isoforms of DSCAM-AS1 in MCF7 cells were identified using 3′ and 5′ RACE ( Fig. 2d and Supplementary Table 1 ). DSCAM-AS1 expression is induced in both MCF7 and T47D cells after oestrogen stimulation, and this induction is reversed with addition of tamoxifen, corroborating that ER is in fact regulating the expression of this lncRNA ( Fig. 2e ). Expression of known ER-regulated protein-coding genes GREB1 and PGR follow the same pattern of response to oestrogen, while the lncRNA MALAT1 , serving as a negative control, is not induced by oestrogen ( Fig. 2e ). In addition to being oestrogen-responsive, DSCAM-AS1 expression is present in both the cytoplasm and nucleus at nearly identical fractions in both MCF7 and T47D cells ( Supplementary Fig. 2d ), and the identity of DSCAM-AS1 as a noncoding gene was corroborated using the CPAT tool [25] ( Supplementary Fig. 2e ). We used single-molecule fluorescence in situ hybridization (ISH) to further dissect the subcellular localization and gene expression levels of DSCSM-AS1 in breast cancer cells. To this end, we designed probes that targeted all potential isoforms of the transcript predicted by RACE. On staining, we found that each MCF7 cell expressed ∼ 800 copies of the DSCAM-AS1 transcript, almost half as much as the expression level of GAPDH ( Supplementary Fig. 2f,g ), additionally the similar nuclear and cytoplasmic localization was corroborated by ISH ( Supplementary Fig. 2h ). While the abundance of DSCAM-AS1 was lower in T47D cells ( ∼ 260 molecules per cell, Supplementary Fig. 2i,j ), the relative expression level (compared with GAPDH) and the subcellular localization pattern were very similar to those observed in MCF7 cells ( Supplementary Fig. 2k ). 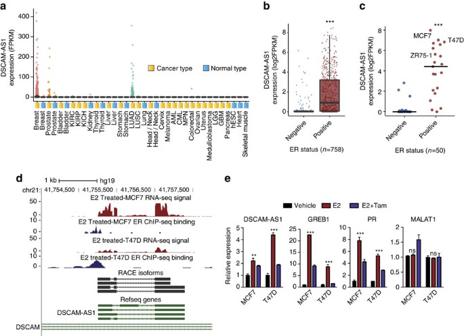Figure 2: Characterization ofDSCAM-AS1. (a) Plot highlighting the expression in FPKM ofDSCAM-AS1in the 6,503 sample MiTranscriptome RNA-seq compendium7categorized by the different cancer/tissue types. Each point represents one RNA-seq tissue sample. (b) Expression ofDSCAM-AS1is significantly higher in ER-positive breast cancer tissue samples (n=584) compared with ER-negative samples (n=174). Expression was analysed in samples for which ER IHC was performed. Each point represents one RNA-seq sample. ***P<0.0001, comparing ER-positive with -negative. (c) Expression ofDSCAM-AS1by RNA-seq in breast cancer cell lines categorized by ER status.DSCAM-AS1expression is significantly higher in ER-positive cell lines (n=21) versus ER-negative cell lines (n=29). Each point represents one cell line. ***P<0.0001, comparing ER-positive to –negative via Student’st-test. (d) UCSC genome browser depiction ofDSCAM-AS1region on chromosome 21. RNA-seq expression track shown in red, and ER ChIP-seq shown in blue. Refseq transcripts shown in green. RACE verified transcript structure shown in black. (e) qPCR expression ofDSCAM-AS1,GREB1,PGR, andMALAT18 h following addition of DMSO vehicle (black), 10 nM estrogen (red), and 10 nM estrogen and 1 μM tamoxifen (blue) in MCF7 and T47D cell lines. Error bars represent s.e.m. for three biological replicates. **P<0.001, ***P<0.0001, NS:P>0.01 comparing with vehicle for each condition via Student’st-test. NS, not significant. Figure 2: Characterization of DSCAM-AS1 . ( a ) Plot highlighting the expression in FPKM of DSCAM-AS1 in the 6,503 sample MiTranscriptome RNA-seq compendium [7] categorized by the different cancer/tissue types. Each point represents one RNA-seq tissue sample. ( b ) Expression of DSCAM-AS1 is significantly higher in ER-positive breast cancer tissue samples ( n =584) compared with ER-negative samples ( n =174). Expression was analysed in samples for which ER IHC was performed. Each point represents one RNA-seq sample. *** P <0.0001, comparing ER-positive with -negative. ( c ) Expression of DSCAM-AS1 by RNA-seq in breast cancer cell lines categorized by ER status. DSCAM-AS1 expression is significantly higher in ER-positive cell lines ( n =21) versus ER-negative cell lines ( n =29). Each point represents one cell line. *** P <0.0001, comparing ER-positive to –negative via Student’s t -test. ( d ) UCSC genome browser depiction of DSCAM-AS1 region on chromosome 21. RNA-seq expression track shown in red, and ER ChIP-seq shown in blue. Refseq transcripts shown in green. RACE verified transcript structure shown in black. ( e ) qPCR expression of DSCAM-AS1 , GREB1 , PGR , and MALAT1 8 h following addition of DMSO vehicle (black), 10 nM estrogen (red), and 10 nM estrogen and 1 μM tamoxifen (blue) in MCF7 and T47D cell lines. Error bars represent s.e.m. for three biological replicates. ** P <0.001, *** P <0.0001, NS: P >0.01 comparing with vehicle for each condition via Student’s t -test. NS, not significant. Full size image DSCAM-AS1 is implicated in cancer aggression We next investigated the clinical relevance of DSCAM-AS1 . Given that DSCAM-AS1 is a lncRNA, its expression is not measured by most traditionally used microarrays, which are the primary high-throughput platforms annotated with reliable clinical outcomes in breast cancer [26] . As a surrogate, we employed a guilt-by-association analysis to interrogate the clinical relevance of those genes most correlated to DSCAM-AS1 . Given that DSCAM-AS1 is an ER-regulated lncRNA, correlation was performed using only ER-positive breast cancers, to ascertain clinical relevance in the breast cancer samples in which DSCAM-AS1 would be enriched and most relevant. We obtained a number of breast cancer clinical data sets from Oncomine [27] containing gene expression sets associated with the presence of cancer (versus normal tissue), high clinical grade, recurrence, survival and metastasis [22] , [23] , [26] , [27] , [28] , [29] , [30] , [31] , [32] , [33] , [34] , [35] , [36] , [37] , [38] , [39] , [40] (Methods section). We assessed for the overlap between these gene sets with the genes most positively or negatively correlated to DSCAM-AS1 . DSCAM-AS1 positively correlated genes were significantly associated with clinical signatures associated with increased cancer aggression, tamoxifen resistance, higher grade, stage and metastasis ( Fig. 3a,b , Supplementary Data 3 and 4 ). Similarly, the DSCAM-AS1 negatively correlated genes associated with clinical signatures that portended a more favourable clinical outcome ( Supplementary Fig. 3a,b , Supplementary Data 3 and 4 ). For many of the clinical concepts, DSCAM-AS1 positively correlated genes displayed a clinical association comparable to those genes most correlated to EZH2 , a gene known to be a marker of clinical aggressiveness in breast cancer [41] , while genes correlated to other lncRNAs expressed in breast tissue, such as HOTAIR, MALAT1 and NEAT1 , showed modest-to-no association ( Fig. 3b , Supplementary Fig. 3b , Supplementary Data 3 and 4 ). In addition, performing a Gene Set Enrichment Analysis (GSEA) [42] on all genes correlated to DSCAM-AS1 yielded significant association with a myriad of breast cancer, cancer aggressiveness, and ER- and tamoxifen-associated gene signatures ( Supplementary Fig. 3c ). While ER-positive breast cancers typically result in better clinical outcomes [23] , among the luminal breast cancers, DSCAM-AS1 is expressed significantly higher in luminal B, a clinical subtype containing most of the clinically aggressive ER-positive breast cancers [22] , [23] ( Fig. 3c ). Despite these associations of clinical aggression with DSCAM-AS1 , in a survival analysis of the ER-positive TCGA breast samples, expression of DSCAM-AS1 was not significantly associated with clinical outcome ( Supplementary Fig. 3d ). Definitive assessment of survival in this cohort, however, will likely require more robust and longer-term clinical curation of the TCGA breast samples. 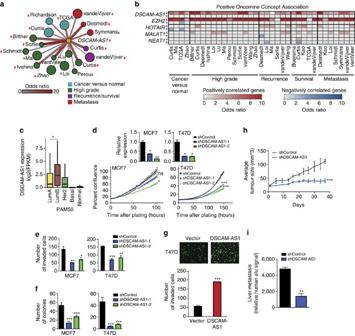Figure 3:DSCAM-AS1is implicated in cancer aggression clinically and in cell lines. (a) Cytoscape depiction of the overlap between the 150 genes most positively correlated withDSCAM-AS1and clinical signatures from Oncomine27for breast cancer clinical outcomes (i.e., recurrence, survival and metastasis), high cancer grade, and cancer versus normal. All significant associations with an odds ratio >6 are shown (Fisher’sPvalue <1E−4). Size of node reflects the size of the gene signature, and the thickness/redness of the line represents the magnitude of the odds ratio. (b) Heatmap displaying the overlap between the top 150 genes correlated toDSCAM-AS1,EZH2,HOTAIR,MALAT1andNEAT1and the genes positively associated with various breast cancer clinical signatures (see above). For each gene, the top row depicts the odds ratio for the positively correlated genes (red), and the bottom row represents the odds ratio for the negatively correlated genes (blue). The first name of the author for each clinical study is listed. (c) Expression ofDSCAM-AS1from breast cancer RNA-seq by PAM50 classification (n=946). Luminal B expression is significantly greater than Luminal A (Student’st-test,P=0.006) (d) Incucyte proliferation assay performed following knockdown ofDSCAM-AS1using two independent shRNAs. Degree of knockdown determined by qPCR shown above. Error bars represent the s.e.m. for three biological replicates. *P<0.01, **P<0.001, ***P<0.0001, NS:P>0.01 comparing to shControl for each condition via Student’st-test. (e) Invasion assay following shRNA knockdown ofDSCAM-AS1using Matrigel coated Boyden chamber assay. Error bars represent the s.e.m. for three biological replicates. *P<0.01, **P<0.001, ***P<0.0001 comparing to shControl for each condition via Student’st-test. (f) Soft agar colony formation assay following shRNA knockdown ofDSCAM-AS1. Error bars represent the s.e.m. for three biological replicates. ***P<0.0001 comparing to shControl for each condition via Student’st-test. (g) Invasion assay following overexpression ofDSCAM-AS1andLacZcontrol. Error bars represent the s.e.m. for three biological replicates. Representative invasion images shown above. ***P<0.0001, comparing to vector overexpression via Student’st-test. (h) Mouse xenograft study of tumour growth for T47D cells with shRNA knockdown ofDSCAM-AS1. Xenografts with shRNA knockdown ofDSCAM-AS1(n=24) exhibited reduced growth when compared to control shRNA knockdown (n=26). Error bars represent the s.e.m. for all xenografts used. ***P<0.0001, comparing to shControl via Student’st-test. (i) Assessment of xenograft metastasis to liver by human Alu PCR, which detects the human cancer cells in the mouse liver. Error bars represent the s.e.m. for three biological replicates. **P<0.001 comparing with shControl via Student’st-test. NS, not significant. Figure 3: DSCAM-AS1 is implicated in cancer aggression clinically and in cell lines. ( a ) Cytoscape depiction of the overlap between the 150 genes most positively correlated with DSCAM-AS1 and clinical signatures from Oncomine [27] for breast cancer clinical outcomes (i.e., recurrence, survival and metastasis), high cancer grade, and cancer versus normal. All significant associations with an odds ratio >6 are shown (Fisher’s P value <1E −4 ). Size of node reflects the size of the gene signature, and the thickness/redness of the line represents the magnitude of the odds ratio. ( b ) Heatmap displaying the overlap between the top 150 genes correlated to DSCAM-AS1 , EZH2 , HOTAIR , MALAT1 and NEAT1 and the genes positively associated with various breast cancer clinical signatures (see above). For each gene, the top row depicts the odds ratio for the positively correlated genes (red), and the bottom row represents the odds ratio for the negatively correlated genes (blue). The first name of the author for each clinical study is listed. ( c ) Expression of DSCAM-AS1 from breast cancer RNA-seq by PAM50 classification ( n =946). Luminal B expression is significantly greater than Luminal A (Student’s t -test, P =0.006) ( d ) Incucyte proliferation assay performed following knockdown of DSCAM-AS1 using two independent shRNAs. Degree of knockdown determined by qPCR shown above. Error bars represent the s.e.m. for three biological replicates. * P <0.01, ** P <0.001, *** P <0.0001, NS: P >0.01 comparing to shControl for each condition via Student’s t -test. ( e ) Invasion assay following shRNA knockdown of DSCAM-AS1 using Matrigel coated Boyden chamber assay. Error bars represent the s.e.m. for three biological replicates. * P <0.01, ** P <0.001, *** P <0.0001 comparing to shControl for each condition via Student’s t -test. ( f ) Soft agar colony formation assay following shRNA knockdown of DSCAM-AS1 . Error bars represent the s.e.m. for three biological replicates. *** P <0.0001 comparing to shControl for each condition via Student’s t -test. ( g ) Invasion assay following overexpression of DSCAM-AS1 and LacZ control. Error bars represent the s.e.m. for three biological replicates. Representative invasion images shown above. *** P <0.0001, comparing to vector overexpression via Student’s t -test. ( h ) Mouse xenograft study of tumour growth for T47D cells with shRNA knockdown of DSCAM-AS1 . Xenografts with shRNA knockdown of DSCAM-AS1 ( n =24) exhibited reduced growth when compared to control shRNA knockdown ( n =26). Error bars represent the s.e.m. for all xenografts used. *** P <0.0001, comparing to shControl via Student’s t -test. ( i ) Assessment of xenograft metastasis to liver by human Alu PCR, which detects the human cancer cells in the mouse liver. Error bars represent the s.e.m. for three biological replicates. ** P <0.001 comparing with shControl via Student’s t -test. NS, not significant. Full size image We then studied the role of DSCAM-AS1 on oncogenic phenotypes in ER-positive breast cancer cell lines. In MCF7 and T47D cells, stable knockdown of DSCAM-AS1 was achieved using shRNA approaches. DSCAM-AS1 knockdown reduced the proliferative ability of both cell lines ( Fig. 3d ), diminished the ability of these cells to invade in a Boyden chamber invasion assay ( Fig. 3e ), and substantially abolished the ability of these cells to form colonies in soft agar ( Fig. 3f ). While ER regulates levels of DSCAM-AS1 , ER expression and protein levels are not dependent on level of DSCAM-AS1 ( Supplementary Fig. 4a ), ruling out the possibility that the phenotype observed could be explained through changes in the level of ER . In addition, knockdown of DSCAM-AS1 exhibited no affect on RNA or protein levels of the DSCAM gene, in which DSCAM-AS1 resides antisense and intronic ( Supplementary Fig. 4b ). To further demonstrate the impact of DSCAM-AS1 on aggressive cancer phenotypes, we overexpressed DSCAM-AS1 in T47D ( Supplementary Fig. 4c ) and ZR75-1 ( Supplementary Fig. 4d ), two ER-positive breast cancer cell lines with moderate DSCAM-AS1 expression ( Fig. 2c ), and observed an increase in the invasion phenotype ( Fig. 3g and Supplementary Fig. 4e ). MCF7 cells were not included in the overexpression studies as DSCAM-AS1 is already expressed at a very high level in these cells ( Fig. 2c ). Overexpression was also tested in MDA-MB-231 cells ( Supplementary Fig. 4f ), a common ER-negative cell line. However, exogenous DSCAM-AS1 was unable to confer oncogenicity via proliferation ( Supplementary Fig. 4g ) and invasion ( Supplementary Fig. 4h ). This phenomenon may be explained by a requisite genetic and epigenetic milieu provided by ER-positive cells in order for DSCAM-AS1 to confer its cancer phenotype, and more investigation into the precise mechanisms through which it acts will shed light on this finding. Furthermore, the simple presence of DSCAM-AS1 alone is not sufficient to make cells highly aggressive, as evidenced by its high expression in ER-positive cell lines that are moderately invasive (for example, MCF7). To further characterize the impact of DSCAM-AS1 on cancer phenotype, we performed a mouse xenograft tumour growth assay, showing that loss of DSCAM-AS1 reduces the growth of implanted T47D cells in vivo ( Fig. 3h ). The metastatic potential of these implanted cells were also reduced with DSCAM-AS1 knockdown, as evidenced through decreased liver metastasis following xenograft ( Fig. 3i ). Role of hnRNPL in DSCAM-AS1 mechanism LncRNAs have been shown to be functional through their binding interactions with other RNAs, DNA, and with proteins [2] . Thus, identifying protein binding partners for DSCAM-AS1 is a crucial step in determining the mechanism through which it confers oncogenicity. To identify DSCAM-AS1 binding partners, we performed pull-down of DSCAM-AS1 and performed mass spectrometry on the pull-down product to identify proteins bound to DSCAM-AS1 ( Fig. 4a ). The protein hnRNPL was observed to have the highest spectral counts for the sense form of DSCAM-AS1 with zero spectral counts in the antisense pull-down ( Fig. 4b ). In addition, PCBP2, a protein known to complex with hnRNPL [43] , was also among the top proteins bound to DSCAM-AS1 . We thus investigated the interaction between DSCAM-AS1 and hnRNPL further. HnRNPL is a protein widely expressed in many tissue types ( Supplementary Fig. 5a ) and has been implicated in regulating RNA stability and processing with subsequent effects on gene expression [44] , [45] , [46] , [47] . The binding of hnRNPL to DSCAM-AS1 was confirmed by RNA pull-down followed by western blot, with no binding of hnRNPL to the negative control antisense transcript ( Fig. 4c ). Other RNA-binding proteins did not bind DSCAM-AS1 , however, suggesting that DSCAM-AS1 does not promiscuously bind to RNA-binding proteins in general ( Fig. 4c ). To further confirm this binding interaction and its specificity, RNA immunoprecipitation (RIP) was performed with using antibodies directed against hnRNPL. DSCAM-AS1 was highly enriched by anti-hnRNPL RIP in both MCF7 and T47D cells, while control coding and noncoding genes exhibited modest binding ( Fig. 4d ). In addition, anti-snRNP70 and anti-HuR RIP failed to pull-down DSCAM-AS1 , further suggesting the specificity of the DSCAM-AS1 -hnRNPL interaction ( Supplementary Fig. 5b ). 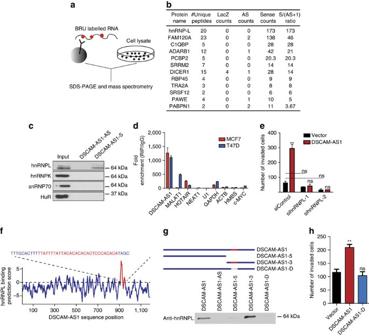Figure 4: Physical and functional relationship ofDSCAM-AS1with hnRNPL. (a) Schematic representation of the RNA pull-down technique used to identify protein binding partners ofDSCAM-AS1. The BRU lableled RNA transcripts are incubated with cell lysate from T47D cells and the eluted protein is resolved by SDS–PAGE. RNA-bound protein product is then processed by mass spectrometry. (b) Top protein binding partners forDSCAM-AS1. Pull-down ofLacZand antisenseDSCAM-AS1used as control. S/AS ratio determined as sense counts divided by 1+antisense counts. (c) Western blot of hnRNPL, hnRNPK, snRNP70, and HuR following pull-down of BRU labelledDSCAM-AS1and antisenseDSCAM-AS1. (d) qPCR following RIP for hnRNPL performed in MCF and T47D cells. Data represented as fold-enrichment over IgG RIP. Error bars represent the s.e.m. for three biological replicates. (e) Invasion assay for T47D cells overexpressingLacZcontrol orDSCAM-AS1following siRNA-mediated knockdown ofhnRNPL. Error bars represent the s.e.m. for two biological replicates. **P<0.001, NS:P>0.01 comparing to siControl (unless otherwise specified with dotted line) for each condition via Student’st-test. (f) Per base in silicoprediction for binding of hnRNPL toDSCAM-AS1.One strong predicted binding peak exists in the 3′ region ofDSCAM-AS1shown in red. (g) Schematic depicting the mutant forms ofDSCAM-AS1generated with or without the predicted binding site (top). Western blot for hnRNPL shown following pull-down of each mutant form ofDSCAM-AS1in HEK293 cells (bottom). (h) Invasion assay in T47D cells overexpressingLacZcontrol, full-lengthDSCAM-AS1, and theDSCAM-AS1-Dmutant. Error bars represent the s.e.m. for three biological replicates. **P<0.001, NS:P>0.01 comparing to vector overexpression for each condition via Student’st-test. NS, not significant; siRNA, small interfering RNA. Figure 4: Physical and functional relationship of DSCAM-AS1 with hnRNPL. ( a ) Schematic representation of the RNA pull-down technique used to identify protein binding partners of DSCAM-AS1 . The BRU lableled RNA transcripts are incubated with cell lysate from T47D cells and the eluted protein is resolved by SDS–PAGE. RNA-bound protein product is then processed by mass spectrometry. ( b ) Top protein binding partners for DSCAM-AS1 . Pull-down of LacZ and antisense DSCAM-AS1 used as control. S/AS ratio determined as sense counts divided by 1+antisense counts. ( c ) Western blot of hnRNPL, hnRNPK, snRNP70, and HuR following pull-down of BRU labelled DSCAM-AS1 and antisense DSCAM-AS1 . ( d ) qPCR following RIP for hnRNPL performed in MCF and T47D cells. Data represented as fold-enrichment over IgG RIP. Error bars represent the s.e.m. for three biological replicates. ( e ) Invasion assay for T47D cells overexpressing LacZ control or DSCAM-AS1 following siRNA-mediated knockdown of hnRNPL . Error bars represent the s.e.m. for two biological replicates. ** P <0.001, NS: P >0.01 comparing to siControl (unless otherwise specified with dotted line) for each condition via Student’s t -test. ( f ) Per base i n silico prediction for binding of hnRNPL to DSCAM-AS1. One strong predicted binding peak exists in the 3′ region of DSCAM-AS1 shown in red. ( g ) Schematic depicting the mutant forms of DSCAM-AS1 generated with or without the predicted binding site (top). Western blot for hnRNPL shown following pull-down of each mutant form of DSCAM-AS1 in HEK293 cells (bottom). ( h ) Invasion assay in T47D cells overexpressing LacZ control, full-length DSCAM-AS1 , and the DSCAM-AS1-D mutant. Error bars represent the s.e.m. for three biological replicates. ** P <0.001, NS: P >0.01 comparing to vector overexpression for each condition via Student’s t -test. NS, not significant; siRNA, small interfering RNA. Full size image To more specifically investigate the functional relationship of DSCAM-AS1 and hnRNPL, we performed rescue studies assessing the impact of hnRNPL knockdown on the invasive advantage conferred by DSCAM-AS1 overexpression, observing that reduction of hnRNPL levels entirely reversed the increase in invasion observed on DSCAM-AS1 overexpression ( Fig. 4e , Supplementary Fig. 6a ). Because there was only slight, non-significant reduction in invasion with hnRNPL knockdown in control cells, the marked reduction in invasion observed in the DSCAM-AS1 overexpressing cells with hnRNPL knockdown may be the result of hnRNPL affecting invasion in a mechanism exclusive to DSCAM-AS1 . So, to further characterize the functional relationship between DSCAM-AS1 and hnRNPL, we set out to localize the binding site of hnRNPL within the DSCAM-AS1 lncRNA. Using in silico prediction drawing from prior studies of hnRNPL crosslinking-immunoprecipitation sequencing (CLIP-seq) [48] , a single strong predicted binding peak was identified near the 3′-end of DSCAM-AS1 ( Fig. 4f ). HnRNPL has been shown to bind CACA-rich RNA sites [45] , and the predicted binding region possessed a 10 base pair CACA stretch. To identify if this predicted region does in fact account for the hnRNPL binding, multiple mutant forms of DSCAM-AS1 were created with or without the binding site. DSCAM-AS1-5 and DSCAM-AS1-3 are large deletion mutants containing only the 5′- and 3′-end, respectively, with only DSCAM-AS1-3 possessing the predicted binding site, and DSCAM-AS1-D is a mutant form with the 27 nucleotides comprising the predicted binding site deleted ( Fig. 4f,g , red). The various mutant forms of DSCAM-AS1 were expressed in HEK293, a cell line that lacks endogenous DSCAM-AS1 expression while still expressing hnRNPL ( Supplementary Fig. 6b ). While both the full-length and DSCAM-AS1-3 mutant retained hnRNPL binding, loss of the predicted binding region was effective in abrogating hnRNPL binding via both Western blot following RNA pull-down ( Fig. 4g ) and by qPCR following hnRNPL RIP ( Supplementary Fig. 6c ). All deletion mutants were expressed at comparable levels, ruling out the possibility of falsely diminished binding due to failed expression of the mutant construct ( Supplementary Fig. 6d ). RNA secondary structure is a crucial component of RNA functionality and is a key player in RNA-protein interactions. While the 27 nucleotide deletion in the DSCAM-AS1-D mutant is a small fraction of the total number of bases in the transcript, to ensure that this deletion was not causing a marked RNA secondary structure change, we investigated the impact of this deletion on RNA secondary structure via the RNAfold structure prediction tool [49] . Evidenced by a minimal free energy prediction, the posited secondary structure of DSCAM-AS1 is largely similar to that of DSCAM-AS1-D ( Supplementary Fig. 6e ), suggesting that the loss of hnRNPL binding observed with the DSCAM-AS1-D mutant is not due to a dramatic secondary structure rearrangement. Quite interestingly, overexpression of the DSCAM-AS1-D mutant in T47D cells failed to recapitulate the increased invasion observed when overexpressing full-length DSCAM-AS1 ( Fig. 4h ). This finding, in combination with the rescue studies following hnRNPL knockdown ( Fig. 4e ), strongly suggest that DSCAM-AS1 promotes oncogenicity via its interaction with hnRNPL in these ER-positive breast cancer cells. Role of DSCAM-AS1 in tamoxifen resistance A substantial number of patients with ER-positive breast cancer eventually develop resistance to endocrine therapy and present with clinical recurrence and metastasis [11] , [50] , [51] . Thus, as DSCAM-AS1 is implicated in poor-prognosis ER-positive breast cancer ( Fig. 3a-c and Supplementary Fig. 3 ), we set out to investigate its potential role in subverting oestrogen dependence and promoting resistance to anti-oestrogen therapies. We continuously passaged MCF7 cells in 1 uM tamoxifen for 6 months until we attained a subpopulation of MCF7 cells that were able to grow in in tamoxifen and termed these tamoxifen-resistant MCF7 cells (TamR-MCF7). Interestingly, although expression of canonical ER targets ( GREB1 and PGR ) was decreased compared to the parental MCF7 cells, DSCAM-AS1 expression was significantly upregulated despite already being expressed at very high levels in MCF7 cells ( Fig. 5a ). The levels of ER were also increased, which is likely a compensatory upregulation in response to the continual anti-oestrogen effects of tamoxifen. Additionally, short-term tamoxifen treatment of parental MCF7 cells transiently reduced DSCAM-AS1 levels at 8hrs following tamoxifen treatment, with a rise back to pre-treatment levels after 24 h ( Supplementary Fig. 7a ). In contrast, canonical ER target, GREB1 , exhibited pronounced expression reduction at both the short- and long-term timescale ( Supplementary Fig. 7b ). To interrogate whether this upregulation of DSCAM-AS1 in the TamR-MCF7 cells is functionally significant, we assessed the proliferative capacity of these cells following DSCAM-AS1 knockdown. With knockdown levels of DSCAM-AS1 comparable to the endogenous levels in parental MCF7 cells ( Supplementary Fig. 7c ), knockdown of DSCAM-AS1 in TamR-MCF7 cells led to a loss of their baseline proliferative advantage when cultured in tamoxifen, exhibiting a proliferation profile nearly identical to that of the parental MCF7 cells ( Fig. 5b ). Additionally, knockdown of hnRNPL in these cells produced a similar loss of proliferative capacity in the TamR-MCF7 cells ( Supplementary Fig. 7d,e ), suggesting that both DSCAM-AS1 and hnRNPL may be playing a role in promotion of the tamoxifen resistance developed by these cells. 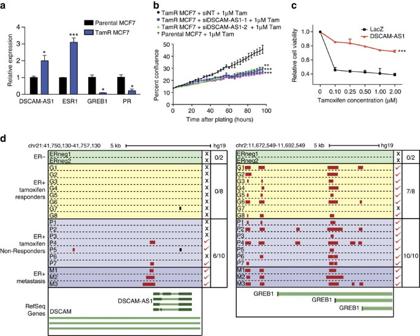Figure 5:DSCAM-AS1is implicated in tamoxifen resistance. (a) qPCR expression ofDSCAM-AS1,ESR1,GREB1andPGRin tamoxifen-resistant MCF7 cells relative to parental MCF7. Error bars represent the s.e.m. for three biological replicates. *P<0.01, ***P<0.0001, comparing to parental MCF7 for each condition via Student’st-test. (b) Proliferation assay in parental MCF7 cells and in TamR-MCF7 cells following siRNA-mediated knockdown ofDSCAM-AS1via two independent siRNAs. Error bars represent the s.e.m. for three biological replicates. **P<0.001, ***P<0.0001, comparing to parental TamR siNT for each condition via Student’st-test. (c) WST viability assay following 10 days of culture in varying levels of tamoxifen performed for T47D cells overexpressing LacZ control andDSCAM-AS1. Error bars represent the s.e.m. for three biological replicates. ***P<0.0001, comparing to LacZ overexpression via Student’st-test. (d) Depiction of oestrogen receptor binding to theDSCAM-AS1(left) andGREB1(right) promoters via ChIP-seq performed in primary and metastatic breast cancer tumour tissues. ER status and response to tamoxifen treatment detailed to left. ER binding peaks (determined using MACS software) are depicted in red (for promoter binding) and black (for non-promoter binding). Promoter defined as 5KB upstream of any transcriptional start site. ER promoter binding indicated by red check or ‘x’ to the right. Genomic coordinates in hg19 listed above. siRNA, small interfering RNA. Figure 5: DSCAM-AS1 is implicated in tamoxifen resistance. ( a ) qPCR expression of DSCAM-AS1 , ESR1 , GREB1 and PGR in tamoxifen-resistant MCF7 cells relative to parental MCF7. Error bars represent the s.e.m. for three biological replicates. * P <0.01, *** P <0.0001, comparing to parental MCF7 for each condition via Student’s t -test. ( b ) Proliferation assay in parental MCF7 cells and in TamR-MCF7 cells following siRNA-mediated knockdown of DSCAM-AS1 via two independent siRNAs. Error bars represent the s.e.m. for three biological replicates. ** P <0.001, *** P <0.0001, comparing to parental TamR siNT for each condition via Student’s t -test. ( c ) WST viability assay following 10 days of culture in varying levels of tamoxifen performed for T47D cells overexpressing LacZ control and DSCAM-AS1 . Error bars represent the s.e.m. for three biological replicates. *** P <0.0001, comparing to LacZ overexpression via Student’s t -test. ( d ) Depiction of oestrogen receptor binding to the DSCAM-AS1 (left) and GREB1 (right) promoters via ChIP-seq performed in primary and metastatic breast cancer tumour tissues. ER status and response to tamoxifen treatment detailed to left. ER binding peaks (determined using MACS software) are depicted in red (for promoter binding) and black (for non-promoter binding). Promoter defined as 5KB upstream of any transcriptional start site. ER promoter binding indicated by red check or ‘x’ to the right. Genomic coordinates in hg19 listed above. siRNA, small interfering RNA. Full size image We also interrogated the ability of DSCAM-AS1 to confer tamoxifen resistance in native T47D cells via overexpression of DSCAM-AS1 . DSCAM-AS1 overexpression was also associated with tamoxifen-resistant growth in a dose-dependent manner, with a striking increase in cell viability at levels of tamoxifen as low was 100 nM ( Fig. 5c ). Additionally, in line with the ability of DSCAM-AS1 to provide oestrogen-independent growth advantage, cells overexpressing DSCAM-AS1 also exhibited a proliferative advantage when grown in oestrogen-deprived medium compared to normal serum ( Supplementary Fig. 7f ). This growth advantage was abolished with the addition of oestrogen, and returned with the subsequent addition of tamoxifen ( Supplementary Fig. 7f ). Conversely corroborating the relationship of DSCAM-AS1 on oestrogen dependence in these cells, we witnessed an increased oestrogen dependence of T47D cells following DSCAM-AS1 knockdown ( Supplementary Fig. 7g ). To corroborate our in vitro findings in a tissue model, we obtained data previously generated performing ChIP-seq for ER in primary and metastatic breast tumour tissue [13] . These tumours were grouped into the following categories as previously described [13] : primary ER-negative ( n =2), primary ER-positive, tamoxifen-responder ( n =8), primary ER-positive, tamoxifen-non-responder ( n =7), metastatic ER-positive ( n =3). Strikingly, investigation of the DSCAM-AS1 promoter revealed that ER preferentially binds to the DSCAM-AS1 promoter in tumours with clinical aggression (ie, metastatic and tamoxifen non-responders; Fig. 5d ), while a canonical ER target, GREB1 , exhibits ER-biding to its promoter in nearly all ER-positive tumours, lacking preference for the more clinically aggressive tumours. Altogether, these data suggest that the association between DSCAM-AS1 expression with clinical aggressiveness in ER-positive breast cancer samples may be explained, in part, by the ability of DSCAM-AS1 to facilitate oestrogen-independent oncogenicity, thus potentially promoting resistance to endocrine therapy with tamoxifen. Further investigation and study of the mechanisms through which ER-dominant breast cancers become aggressive and eventually evade traditional clinical therapies is of intense clinical interest. In this study, we identify a myriad of potentially ER-associated lncRNAs, and functionally and mechanistically characterize one of the most intriguing candidates. Nevertheless, further investigation of some of these other lncRNAs may also contribute to our understanding of ER biology and ER-driven oncogenesis. LncRNAs have been shown to function through multiple mechanisms, and the study of the interaction of DSCAM-AS1 with hnRNPL is a promising step towards understanding the ways through which this molecule executes its oncogenic function. While we show that the binding of hnRNPL to DSCAM-AS1 is responsible for at least some of its oncogenicity, a further understanding of how the interaction between hnRNPL and DSCAM-AS1 is mediating this phenotype is necessary. Novel mediators of tumour aggression, such as DSCAM-AS1 , can provide insight into the mechanism of endocrine therapy resistance. This increased understanding may in turn lead to more effective strategies to overcome this resistance, which is one of the last, great clinical challenges in treatment of ER-positive breast cancer. In addition, there is little known regarding the role of noncoding RNAs in developing resistance to anti-oestrogen therapy, with a small number of studies implicating some of the more prominent, well characterized breast cancer lncRNAs [52] , [53] . DSCAM-AS1 is just one of many potentially relevant ER-regulated lncRNAs in breast cancer, and further investigation of the other candidates is likely to yield a greater understanding of ER-mediated cancer biology. Ultimately, this study provides key insight into the role of lncRNAs in ER breast cancer biology, and is an important step in better understanding this common disease. Cell lines and cell culture All cell lines were obtained from the American Type Culture Collection (Manassas, VA). Cell lines were maintained using standard media and conditions. Specifically, T47D cells were maintained in Roswell Park Memorial Institute (RPMI) 1640 medium supplemented with 10% fetal bovine serum, 1% penicillin-streptomycin and 5 mg ml −1 insulin. ZR75-1 cells were maintained in RPMI 1640 medium supplemented with 10% fetal bovine serum, 1% penicillin-streptomycin. HEK293 cells were maintained in DMEM plus 10% fetal bovine serum (FBS) plus 1% penicillin-streptomycin. MCF7 cells were cultured in Dulbecco’s modified Eagle’s medium plus GlutaMAX (DMEM, Invitrogen) containing 10% fetal bovine serum (Hyclone) and 1% penicillin-streptomycin. To establish the tamoxifen-resistant cell line, MCF7 cells were grown in IMEM phenol-red free medium with 10% Charcoal-stripped FBS in the presence of 1 uM (Z)-4-hydroxytamoxifen (Sigma) for 6 months. All cell lines were grown at 37 °C in a 5% CO 2 cell culture incubator, and were genotyped for identity at the University of Michigan Sequencing Core and tested routinely for Mycoplasma contamination. Cell proliferation assay Cells were seeded in a 48-well plate at 3 × 10 4 cells per well. Plates were added to Incucyte machine (Essen Bioscience) 16–20 h following seeding. Growth curves were constructed by imaging plates using the Incucyte system, where the growth curves are generated from confluence measurements acquired during continuous kinetic imaging. Four wells were measured per condition. For tamoxifen treatment, 16–20 h after seeding, the medium was changed to RPMI phenol-red free medium containing 10% charcoal-treated FBS in the presence of 1 uM tamoxifen or ethanol. Growth curves were obtained using Incucyte system as described above. Cell viability assay Cells were seeded in 96-well plates at 5,000 cells per well in a total volume of 100 μl media containing 10% FBS. Serially diluted tamoxifen in 100 μl of media was added to the cells 12 h after seeding. Medium containing tamoxifen was replenished every 2–3 days. Following 10 days of incubation, cell viability was assessed by WST assay (WST-8, Dojindo). All assays were performed in triplicate and repeated at least three times. The relative cell viability was expressed as a percentage of the control that was treated with vehicle solutions. Soft agar colony formation assay 10,000 cells were suspended in medium containing 0.3% agar, 10% FBS, and layered on medium containing 0.6% agar and 10% FBS in six-well plate. Colonies were stained for 18–24 h with iodonitrotetrozolium chloride (Sigma #18377) following 3 weeks of incubation. Colonies from three replicate wells were quantified. Quantitative RT–PCR assay The miRNeasy mini kit was utilized to isolate RNA from cell lysates. From 1 μg of isolated RNA, SuperScript III (Invitrogen) and Random Primers (Invitrogen) were used to generate cDNA according to the manufacturer's protocol. The ABI7900 HT Fast Real time system (Applied Biosystems) was utilized for quantitiative reverse transcriptase–PCR (qRT–PCR) reactions. Gene-specific primer were designed using the Primer3 software and were subsequently synthesized by IDT Technologies. A relative quantification method was used in analysing the qRT–PCR data and data were depicted as average fold change versus the control (as internal reference, GAPDH and actin were utilized). All primers used for qPCR are detailed in Supplementary Table 2 . Three technical replicates were used in each assay, and all data shown was performed with at least three biological replicates. Oestrogen and tamoxifen treatment To evaluate the effect of oestrogen stimulation, cells were first hormone depleted via growth in phenol-red free medium containing 10% charcoal-treated FBS for 72 h and then treated with ethanol vehicle, 10 nM β-estradiol, or 10 nM β-estradiol plus 1 uM tamoxifen. After 10 h, RNA was isolated as described above and qPCR was performed as described above using Power SYBR Green Mastermix (Applied Biosystems). Subcellular fractionation Cellular fractionation was performed using a RiboTrap Kit (MBL International), according to manufacturer’s instructions. RNA was isolated and qRT–PCR was performed as described above. Knockdown and overexpression studies Knockdown of DSCAM-AS1 and hnRNPL in T47D and MCF7 cells was accomplished by small interfering RNA from Dharmacon. Transfections were performed with OptiMEM (Invitrogen) and RNAi Max (Invitrogen) per manufacturer instruction. Target sequences used for shRNA or small interfering RNA knockdown are listed in Supplementary Table 3 . For stable knockdown of DSCAM-AS1 , MCF7 and T47D cells were transfected with lentiviral constructs containing 2 different DSCAM-AS1 shRNAs or no targeting shRNAs in the presence of polybrene (8 μg ml −1 Supplementary Table 3 ). After 48 h, transduced cells were grown in culture media containing 2 μg ml −1 puromycin. For DSCAM-AS1 overexpression, the predominant isoform (isoform 2, Supplementary Table 1 ) was cloned into the pLenti6.3 vector (Invitrogen) using PCR8 non-directional Gateway cloning (Invitrogen) as an initial cloning vector and shuttling was then done to pLenti6.3 using LR clonase II (Invitrogen) according to the manufacturer's instructions. As control, LacZ was also cloned into the same vector system. The primers for making DSCAM-AS1 mutation and truncations are listed in Supplementary Table 2 . Lentiviral particles were made and T47D and ZR75.1 cells were transduced as described above. Stable cell lines were generated by selection with 3 μg ml −1 blasticidin. Transient transfection of DSCAM-AS1 and its derivative mutants was done in HEK293 cells was performed with Lipofectamine LTX (Invitrogen) following manufacturer’s instruction. Cells were collected at 48 h post transfection. In vitro RNA-binding assay The RNA-binding assay was performed according to the protocol of the RiboTrap Kit (MBL International). In brief, 5-bromo-UTP (BrU) was randomly incorporated into sense DSCAM-AS1 , antisense DSCAM-AS1 , and LacZ control via PCR-based transcription. The primers are shown in Supplementary Table 2 . The the BrU labelled RNA transcripts were bound to beads conjugated with anti-BrdU antibodies. Then, the cytoplasmic or nuclear fractions from MCF7 or T47D cells were mixed for 2 h. Samples were washed four times with Wash Buffer II before elution. The samples were sent to the Michigan Center for Translational Pathology proteomic core facility for mass spectrometry. Mass spectrometry The samples were treated with SDS-PAGE loading buffer supplied with 10 mM DTT for 5 min at 85 °C. The proteins were alkylated by the addition of iodoacetamide to the final concentration of 15 mM. The samples were subjected to SDS–PAGE and the whole lanes were cut out and digested with trypsin in-gel for 2 h. The resulting peptides were extracted, dried and resuspended in 0.1% formic acid with 5% acetonitrile before loading onto a 2 cm EASY-column (Thermo Scientific) coupled to an in-house made nano HPLC column (20 cm × 75 um) packed with LUNA C18 media (Phenomenex). Analysis was performed on a Velos Pro mass spectrometer (Thermo Scientific) operated in data-dependent mode using 120-min gradients in EASY-LC system (Proxeon) with 95% water, 5% acetonitrile (ACN), 0.1% formic acid (FA) (solvent A), and 95% ACN, 5% water, 0.1% FA (solvent B) at a flow rate of 220 nl min −1 . The acquisition cycle consisted of a survey MS scan in the normal mode followed by 12 data-dependent MS/MS scans acquired in the rapid mode. Charge state was not recorded. Dynamic exclusion was used with the following parameters: exclusion size 500, repeat count 1, repeat duration 10 s, exclusion time 45 s. Target value was set at 10 4 for tandem MS scan. The precursor isolation window was set at 2 m/z . The complete analysis comprised two independent biological replicates. Mass spectrometry data analysis The resulting spectrum files were transformed into MGF format by MSConvert software and interrogated by MASCOT 2.4 search engine using human UniProt database version 15 concatenated with reverse sequences for estimation of false discovery rate (FDR) and with a list of common contaminants (40,729 entries in total). The search parameters were as follows: full tryptic search, 2 allowed missed cleavages, peptide charges +2 and +3 only, MS tolerance 1 Da, MS/MS tolerance 0.5 Da. Permanent post-translational modification was: cysteine carbamidomethylation. Variable post-translational modifications were: protein N-terminal acetylation, Met oxidation and N-terminal Glutamine to pyro-Glutamate conversion. The remaining analysis was performed as previously described [54] . To summarize, the minimal ion score threshold was chosen such that a peptide FDR below 1% was achieved. The peptide FDR was calculated as: 2 × (decoy_hits)/(target+decoy hits). The mass spectrometry proteomics data have been deposited to the ProteomeXchange Consortium [55] via the PRIDE partner repository with the data set identifier PXD002421 and 10.6019/PXD002421. Spectral counts for all detected proteins were assembled using an in-house written Python script. The adjustment of spectral counts was done as previously described [54] . RNA immunoprecipitation RIP assays were performed using a Millipore EZ-Magna RIP RNA-Binding Protein Immunoprecipitation kit (Millipore, #17-700) according to the manufacturer's instructions. RIP-PCR was performed as qPCR, as described above, using total RNA as input controls. 1:150th of RIP RNA product was used per PCR reaction. Antibodies used for RIP are listed in Supplementary Table 4 . All RIP assays were performed in biological duplicate. Invasion assay 3 × 10 5 cells were seeded in a 24-well corning FluoroBlok chamber pre-coated with Matrigel (BD Biosciences). Medium containing 10% FBS in the lower chamber served as chemoattractant. After 48 h, cells remaining on the lower side of the membrane were stained with calcein AM (C34852 invitrogen). The invasive cells adhering to the bottom surface of the filter were quantified under a fluorescent microscope (× 2). Antibodies and immunoblot analyses Western immunoblot assays were performed by running cell lysates on 4–12% SDS polyacrylamide gels (Novex) to separate proteins. Proteins were then transferred to a nitrocellulose membrane (Novex) via wet transfer at 30 V overnight. Blocking buffer incubation was then performed for 1 h (Tris-buffered saline, 0.1% Tween (TBS-T), 5% nonfat dry milk). Indicated antibodies were then added to membrane and incubated at 4 °C overnight. Enhanced chemiluminescence (ECL Prime) was utilized to develop blots via the manufacturer's protocol. All the antibodies used in this study are described in Supplementary Table 4 . Representative full blot images are shown in Supplementary Fig. 8 . Chromatin immunoprecipitation HighCell# ChIP kit (Diagenode) was utilized to perform ChIP assays via the manufacturer's protocol. Briefly, MCF7 cells were grown in charcoal-stripped serum media (described above) for 72 h and then stimulated 10 nM estradiol for 12 h. Cells were then crosslinked using 1% formaldehyde for 10 min, and crosslinking was quenched for 5 min at room temperature using a 1/10 volume of 1.25 M glycine. Cells were then lysed and sonicated (Bioruptor, Diagenode), yielding an average chromatin fragment size of 300 bp. An equivalent amount of chromatin equivalent to 5 × 10 6 cells was used for the ChIP for all antibodies. DNA bound to immunoprecipitated product was isolated (IPure Kit, Diagenode) via overnight incubation with antibody at 4 °C. Samples were then washed, and crosslinked reversed. ChIP-seq library construction and sequencing analysis DNA was purified for library preparation using the IPure Kit (Diagenode). The ChIP-seq sample preparation for sequencing was performed according to the manufacturer's instructions (Illumina). ChIP-enriched DNA samples (1–10 ng) were converted into blunt-ended fragments using T4 DNA polymerase, Escherichia coli DNA polymerase I large fragment (Klenow polymerase) and T4 polynucleotide kinase (New England BioLabs (NEB)). A single adenine base was added to fragment ends by Klenow fragment (3′ to 5′ exo − ; NEB) followed by ligation of Illumina adaptors (Quick ligase, NEB). The adaptor-modified DNA fragments were enriched by PCR using the Illumina Barcode primers and Phusion DNA polymerase (NEB). PCR products were size selected using 3% NuSieve agarose gels (Lonza) followed by gel extraction using QIAEX II reagents (QIAGEN). Libraries were quantified with the Bioanalyzer 2100 (Agilent) and sequenced on the Illumina HiSeq 2000 Sequencer (100-nucleotide read length). ChIP-seq data were mapped to human genome version hg19 using BWA [56] . The MACS program [57] was used to generate coverage map files to visualize the raw signal on the UCSC genome browser [58] . Hpeak [59] , a hidden Markov model (HMM)-based peak-calling software program designed for the identification of protein-interactive genomic regions, was used for ChIP-seq peak determination. ChIP-seq peak promoter overlap Overlap of ChIP-seq peaks with gene promoters was performed using the BEDTools ‘coverage’ tool. Intervals of ±5–10 kilobases surrounding unique transcriptional starts were used to assess promoter overlap. Coding potential scoring Coding potential for all lncRNA transcripts was determined as described previously [4] . The alignment-free Coding Potential Assessment Tool (CPAT) [25] was used to determine coding probability for each transcript. CPAT determines the coding probability of transcript sequences using a logistic regression model built from ORF size, Fickett TESTCODE statistic, and hexamer usage bias. Xenograft analysis All experimental procedures were approved by the University of Michigan Committee for the Use and Care of Animals (UCUCA) and conform to all regulatory standards. A total of 5 × 10 6 cells of T47D control or T47D shM41 cells were suspended in 100 ul of PBS/Matrigel (1:1) were injected subcutaneously in 5-week-old pathogen-free female CB-17 severe combine immunodefiecient mice (CB-17 SCID) which simultaneously received a 60-day slow release pellet containing 0.18 mg of 17b-estradiol (Innovative Research of America). Tumours were measured weekly using a digital caliper. Growth in tumour volume was recorded using digital calipers and tumour volumes were estimated using the formula (π/6) ( L × W 2 ), where L =length of tumour and W =width. In addition, mouse livers were collected to determine spontaneous metastasis by measuring human Alu sequence. Briefly, genomic DNA from livers were prepared using Puregene DNA purification system (Qiagen), followed by quantification of human Alu sequence by human Alu specific Fluorogenic Taqman qPCR probes. RNA-seq data processing Sequence quality control was done using FASTQC ( http://www.bioinformatics.babraham.ac.uk/projects/fastqc ). Next, reads mapping to mitochondrial DNA, ribosomal RNA, poly-A, poly-C, Illumina sequencing adaptors, and the spiked-in phiX174 viral genome were filtered. Sequences were downloaded from the Illumina iGenomes server (2012, March 9). Mapping was performed using bowtie2 (2.0.2). Reads were mapped using TopHat2 (2.0.6 and 2.0.8) using default parameters. A human genome reference was constructed from UCSC version Feb 2009 (GRCh37/hg19) chromosomes 1–22, X, Y and mitochondrial DNA, and references from alternate haplotype alleles were omitted. Bowtie-build and bowtie2-build were used to build genome reference for Bowtie versions 0.12.8 and 2.0.2 were, respectively. The Ensembl version 69 transcriptome was used as a reference gene set. Using the --transcriptome-index option in TopHat version 2.0.6 (ref. 60 ), alignment index files were prepared from this reference for Bowtie versions 0.12.8 and 2.0.2. RNA-seq transcript expression estimation Cufflinks version 2.1.1 (ref. 61 ) was used with the following parameters to estimate transcript abundance from RNA-seq data: ‘--max-frag-multihits=1’, ‘--no-effective-length-correction’, ‘--max-bundle-length 5000000’, ‘--max-bundle-frags 20000000’. To convert FPKM abundance estimates (generated by Cufflinks) to approximate fragment count values we multiplied each FPKM by the transcript length (in kilobases) and by the ‘Map Mass’ value (divided by 1.0E 6 ) found in the Cufflinks log files. Breast cancer tissue expression heatmap generation The ‘gplots’ R-package was used to generate heatmaps using the heatmap.2 function. For the cancer versus normal heatmap, expression was normalized as log2 of the fold change over the median of the normal samples for each transcript. For the ER-positive versus ER-negative heatmap, expression was normalized to the median of the ER-negative samples. Unsupervised heirarchical clustering was performed with the hclust function, using Pearson correlation as the clustering distance, using the ‘ward’ agglomeration method. RNA-seq differential expression testing Differential expression testing was performed using the SSEA tool described previously [7] . Briefly, following count data normalization, SSEA performs the weighted KS-test procedure described in GSEA [42] . The resulting enrichment score statistic describes the enrichment of the sample set among all samples being tested. To test for significance, SSEA enrichment tests are performed following random shuffling of the sample labels. These shuffled enrichment tests are used to derive a set of null enrichment scores (1,000 null enrichment scores computed). The nominal P value reported is the relative rank of the observed enrichment score within the null enrichment scores. Multiple hypothesis testing is performed by comparing the enrichment score of the test to the null normalized enrichment score distributions for all transcripts in a sample set. This null normalized enrichment score distribution is used to compute FDR Q values in the same manner used by GSEA [42] . Associations with oncomine clinical signatures We identified the top 150 positively and negatively correlated genes (Spearman’s correlation) to DSCAM-AS1 among the ER-positive breast cancer samples. These gene lists were imported into Oncomine [27] as custom concepts. We then nominated significantly associated breast cancer concepts with odds ratio >4.0 for negatively associated concepts and >6.0 for positively associated concepts and P value <1 × 10 −6 . Nodes and edges of these associations were exported and a concept association network was generated using Cytoscape version 3.2.1. Node positions were computed using the Force-Directed Layout algorithm in Cytoscape using the odds ratio as the edge weight. Node positions were subtly altered manually to enable better visualization of node labels. Association of correlation signatures with oncomine concepts Correlation analysis described above was performed for DSCAM-AS1 , EZH2 , HOTAIR , MALAT1 , and NEAT1 . For each gene, we created a signature of the top 150 most positively and top 150 most negatively correlated genes. We performed a Fisher’s exact test of overlap for each of the above gene signatures with Oncomine clinical signatures for cancer versus normal, clinical recurrence, clinical survival, metastasis, and high clinical grade. The following studies were utilized: Curtis Breast [26] , Ma Breas [62] , TCGA Breast [28] , Zhao Breast [29] , Bittner Breast [63] , Desmedt Breast [30] , Ivshina Breast [31] , Loi Breast [32] , Lu Breast [33] , Perou Breast [22] , Schmidt Breast [34] , Sorlie Breast [23] , vantVeer Breast [64] , Wang Breast [36] , Boersma Breast [37] , Kao Breast [38] , Symmans Breast [39] and vandeVijver Breast [40] . For each Oncomine concept, overlap was tested for the top 1, 5 and 10% of genes up- and downregulated, and the gene signature with the greatest odds ratio was selected for each study. Signature comparisons were performed using a one-sided Fisher's exact test. Survival analysis with TCGA breast data Association of DSCAM-AS1 levels on clinical outcomes was assessed using the TCGA breast cohort. Survival data was obtained from the TCGA data portal. ER-positive samples were used for survival analysis as indicated by the TCGA clinical metadata via IHC status. Samples with DSCAM-AS1 expression >10 FPKM were grouped into the ‘DSCAM-AS1 high’ category and samples with expression <1 FPKM were grouped into the ‘DSCAM-AS1 low’ category. Kaplan-Meier analysis was performed, and log-rank test was performed to assess statistical significance. Tissue expression level percentile metric To generate a metric to summarize the expression of each lncRNA in breast cancer tissues, we identified the expression level of the 95th percentile sample among all breast RNA-seq samples including cancers tissue, normal tissue, and cell lines. RNA-sequencing library preparation Total RNA was obtained from cancer cell lines, and RNA quality was determined using an Agilent Bioanalyzer. Poly-A transcriptome libraries from the mRNA fractions were generated following the Illumina RNA-seq protocol. Each sample was sequenced in a single lane with the Illumina HiSeq 2000 (100-nucleotide read length) as previously described [3] , [65] . The dUTP method of second-strand marking was used for strand-specific library preparation as described previously [66] . Gene set enrichment analysis Expression levels of DSCAM-AS1 were correlated (Spearman) to the expression of all protein-coding genes across all ER-positive breast cancers. The protein-coding genes were then ranked by the Spearman Rho value, and used in a weighted, preranked GSEA analysis against MSigDB gene sets V5.0 (ref. 67 ). In silico binding prediction To obtain potential HNRNPL binding sites on DSCAM-AS1, we utilized GraphProt [68] to learn a predictive model from genome-wide HNRNPL binding sites identified by iCLIP-seq [48] . For training data generation, we extracted the genomic binding positions (GSE37560) with BED table scores >=10, followed by an extension of ±20 nt resulting in 41 nt long binding sites. After mapping the sites to annotated RefSeq genes obtained from UCSC, an equally-sized set of negative sites was selected such that the sites were on the same RefSeq genes and did not overlap with any of the identified positive sites from the initial table. The GraphProt sequence model trained on these data was then used to identify high-scoring sites in the DSCAM-AS1 sequence (NCBI GenBank NR_038899.1). The highest-scoring site centred at RNA position 923 contains a CA-repeat motif known for its affinity towards HNRNPL and was thus used for subsequent analysis. Rapid amplification of cDNA ends (RACE) 5′ and 3′ RACE was performed using the GeneRacer RLM-RACE kit (Invitrogen) according to the manufacturer’s protocols. RACE PCR products obtained using Platinum Taq high-fidelity polymerase (Invitrogen), were resolved on a 1.5% agarose gel. Individual bands were gel purified using a Gel Extraction kit (Qiagen), and cloned into PCR4 TOPO vector, and sequenced using M13 primers. Single-molecule fluorescence in situ hybridization Single-molecule fluorescence in situ hybridization was performed as described [69] , with some minor modifications. Cells were grown on 8-well chambered coverglasses, formaldehyde fixed and permeablized overnight at 4 o C using 70% ethanol. Cells were rehydrated in a solution containing 10% formamide and 2 × SSC for 5 min and then treated with 10 nM fluorescence in situ hybridization probes for 16 h in 2 × SSC containing 10% dextran sulfate, 2 mM vanadyl-ribonucleoside complex, 0.02% RNAse-free BSA, 1 μg μl −1 E. coli transfer RNA and 10% formamide at 37 °C. After hybridization, cells were washed twice for 30 min at 37 °C using a wash buffer (10% formamide in 2 × SSC). Cells were then mounted in solution containing 10 mM Tris/HCl pH 7.5, 2 × SSC, 2 mM trolox, 50 μM protocatechiuc acid and 50 nM protocatechuate dehydrogenase. fluorescence in situ hybridization samples were imaged in three dimensions using HILO illumination as described [70] . Images were processed using custom-written macros in ImageJ. Analysis routines comprises 3 major steps: background subtraction, Laplacian of Gaussian (LoG) filtering and thresholding. Spots with intensity above set threshold are represented in images. Probes were designed to target all isoforms of the DSCAM-AS1 transcript. Probe sequences targeting DSCAM-AS1 (21 probes per transcript) are as follows: 5′-cctatccctttctctaagaa-3′, 5′-acttctgcaaaaacgtgctg-3′, 5′-ggttccactccattttaatt-3′, 5′-ctatagcgtcttatcagctg-3′, 5′-catgtgtccggatatcattt-3′, 5′-tcagtgagtggataactggt-3′, 5′-aattctagtggaggcaccta-3′, 5′-ctaagtagcttcatctttcc-3′, 5′-caactgcgtgtttcctagtc-3′, 5′-agcattctctgttttaacca-3′, 5′-ttagcaactgccttgctctg-3′, 5′-gctgtccagttttagtaaca-3′, 5′-cgttgtgagcctgagagatc-3′, 5′-agaacttccctagaggagtg-3′, 5′-atggggagtgagaccaaaca-3′, 5′-tggaggagggacagagaagg, 5′-tgtgggtgattggtactttt-3′, 5′-atggatgagtatgtcatgcc-3′, 5′-tattgccatggttagcatga-3′, 5′-aatgcatgcttgatggagct-3′. Data availability Sequence data that support the findings of this study have been deposited in the Short Read Archive with the accession code SRP078392. Tissue ChIP-seq data referenced in this study are available in the Gene Expression Omnibus with the accession code GSE32222. All remaining data are contained within the Article and Supplementary Information files or available from the author on request. How to cite this article: Niknafs, Y. S. et al. The lncRNA landscape of breast cancer reveals a role for DSCAM-AS1 in breast cancer progression. Nat. Commun. 7:12791 doi: 10.1038/ncomms12791 (2016).